Controlled charge trapping by molybdenum disulphide and graphene in ultrathin heterostructured memory devices Atomically thin two-dimensional materials have emerged as promising candidates for flexible and transparent electronic applications. Here we show non-volatile memory devices, based on field-effect transistors with large hysteresis, consisting entirely of stacked two-dimensional materials. Graphene and molybdenum disulphide were employed as both channel and charge-trapping layers, whereas hexagonal boron nitride was used as a tunnel barrier. In these ultrathin heterostructured memory devices, the atomically thin molybdenum disulphide or graphene-trapping layer stores charge tunnelled through hexagonal boron nitride, serving as a floating gate to control the charge transport in the graphene or molybdenum disulphide channel. By varying the thicknesses of two-dimensional materials and modifying the stacking order, the hysteresis and conductance polarity of the field-effect transistor can be controlled. These devices show high mobility, high on/off current ratio, large memory window and stable retention, providing a promising route towards flexible and transparent memory devices utilizing atomically thin two-dimensional materials. The remarkable properties of graphene, such as high carrier mobility, thermal conductivity, mechanical flexibility and optical transparency, make it a highly promising material for future electronics [1] , [2] . The ongoing development of graphene electronics has been accompanied by increasing interest in other two-dimensional (2D) layered materials with different electronic properties, which can be combined with graphene into other layered heterostructures [3] , [4] , [5] , [6] . For instance, insulating hexagonal boron nitride (hBN) has emerged as an excellent substrate for graphene, yielding graphene devices with improved mobility and lower disorder compared with more conventional dielectrics [4] . Furthermore, hBN is atomically flat and, thus, it can serve as a uniform tunnelling barrier that allows perfectly planar charge injection [7] . Semiconducting molybdenum disulphide (MoS 2 ), another 2D material, shows a transition from an indirect band gap of 1.3 eV in the bulk to a direct band gap of 1.8 eV for a monolayer [6] . MoS 2 field-effect transistors (FETs) with high mobility (200 cm 2 V −1 s −1 ) and an on/off ratio of ~10 8 have also been recently reported [5] . Such excellent electrical properties, high transparency and flexibility, altogether make these 2D materials perfect candidates for flexible electronics. Moreover, rapid development in the synthesis of 2D materials is improving prospects for mass production and large-scale integration of 2D electronic materials [1] , [8] , [9] , [10] , [11] , [12] . Multi-stacking of atomically thin 2D materials enables vertical integration and use of conventional lithography process. Recently, heterostructure of 2D materials produced by multi-stacking process opened up a route to make new types of material platforms for high-performance devices [4] , [13] , [14] , [15] . A number of reports have utilized graphene or graphene oxide in non-volatile memory devices, such as an FET channel, a charge-trapping layer or an electrode [16] , [17] , [18] , [19] , [20] , [21] , [22] . It was shown that the large hysteresis in the gate characterization curves of graphene FETs (GFETs) can be applied for memory device operation [23] . It was also demonstrated that this hysteresis arises due to trapped charge in the oxide dielectric layer [24] . However, the relatively slow dynamics and poor controllability of the trap density in these graphene memory devices require further improvement for realistic applications. Furthermore, insulator (or tunnel barrier) and channel material with band gap, which should be ultrathin and stable, have been required for flexible and transparent memory applications. In this sense, the 2D materials, such as hBN and MoS 2 , can be great candidates thanks to their superior electrical and mechanical properties [4] , [7] , [25] . Here we demonstrate memory devices fabricated entirely from stacked 2D materials. We fabricated two types of 2D heterostructured memory devices, which show a significant hysteresis and memory performance thanks to the charge-trapping characteristics of graphene and MoS 2 . One of the two types of the memory devices was fabricated with graphene as the FET channel, hBN as the tunnel barrier and MoS 2 as the charge-trapping layer (denoted as GBM) and the other with MoS 2 as the FET channel, hBN as the tunnel barrier and graphene as the charge trapping layer (denoted as MBG). These ultrathin heterostructured memory devices (thinner than 10 nm) consisting of 2D materials has great potential for further miniaturization, application in low-cost electronics and flexible memory device applications, especially in the future mobile devices requiring embedded memories integrated into multi-functional system-on-a-chip. Memory characteristics of heterostructured devices Heterostructured devices were fabricated by stacking 2D materials, which are prepared by mechanical exfoliation (see Methods and Supplementary Fig. S1 ) In the case of GBM devices, to verify the effect of charge trapping in MoS 2 , the graphene sample was cut into two regions—one region with and the other without MoS 2 . 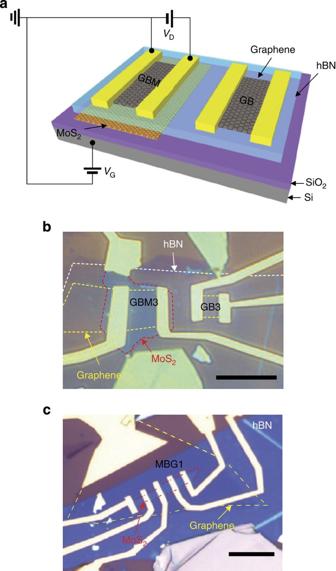Figure 1: Structure of heterostructured memory devices. (a) Schematic and circuit diagram of the fabricated device. Optical micrographs of (b) GBM and (c) MBG devices. Scale bars, 10 μm. The devices ofbandcare denoted as GBM3, GB3 and MBG1, respectively. The dotted lines indicate the boundaries of each 2D material. Figure 1a shows the circuit diagram of a fabricated GBM device. Figure 1b shows optical micrographs of GBM and MBG devices. In Fig. 1b , a graphene/hBN device without MoS 2 is denoted as GB. Supplementary Fig. S2 and Supplementary Table S1 summarize the Raman spectra and photoluminescence (PL) of graphene, hBN, MoS 2 layers and thickness of each layer of the devices fabricated for this study. Figure 1: Structure of heterostructured memory devices. ( a ) Schematic and circuit diagram of the fabricated device. Optical micrographs of ( b ) GBM and ( c ) MBG devices. Scale bars, 10 μm. The devices of b and c are denoted as GBM3, GB3 and MBG1, respectively. The dotted lines indicate the boundaries of each 2D material. 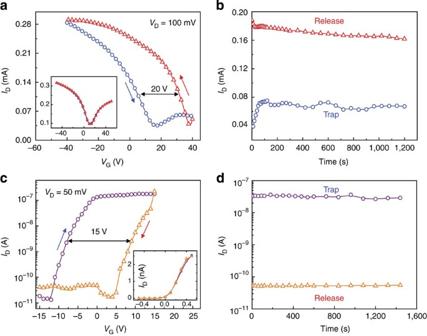Figure 2: Transfer and retention characteristics of heterostructured devices. (a) Transfer curve (ID−VG) and (b) retention performance of the GBM3 device with hBN of 6 nm and MoS2of 5 nm. The inset ofashows a transfer curve of GB3. For GBM devices, all the transfer curves in the main text were obtained atVD=100 mV and medium sweep rate of 23 V s−1. The retention ofbwas measured atVG=15 V with a pulse of +40 V (red triangle) and −40 V (blue circle), pulse width of 1 ms andVD=100 mV. (c) Transfer curve and (d) retention performance of the MBG1 device with hBN of 12 nm, MoS2of three layers and graphene of two layers. The inset ofcshows a transfer curve of the same device when graphene was used for gating. For MBG devices, all the measurement of transfer curve in the main text was obtained atVD=50 mV and medium sweep rate of 23 V s−1. The retention ofdwas measured atVG=0 V with pulse of −15 V (violet circle) and +15 V (orange triangle), pulse width of 100 μs andVD=50 mV. Full size image Figure 2a shows the transfer curve of one device (GBM3), with an hBN layer of 6 nm thick and a MoS 2 layer of 5 nm thick. The position of the Dirac point, corresponding to the minimum conductivity, shifts by more than 20 V and exhibits a large hysteresis when the direction of the gate voltage sweep is reversed. This remarkable hysteresis is related to underlying MoS 2 layer, as there is no appreciable hysteresis in the transfer curve of GB3, a graphene device on the same graphene sample as GBM3 but without underlying MoS 2 layer, as shown in the inset of Fig. 2a . The field-effect mobility of graphene in GBM3 is 4,200 cm 2 V −1 s −1 , which is lower than reported in graphene on hBN [4] . This mobility degradation is likely due to the presence of a small number of bubbles and wrinkles, as observed in the atomic force microscopy images of Supplementary Fig. S3 , which can introduce charge inhomogeneity [26] . However, as hysteresis is not observed in all the GB devices, it is obvious that the existence of underlying MoS 2 layer gives rise to the hysteresis in transfer curve of the GBM devices. Even when different voltage sweep rates are applied, no appreciable differences are noted in transfer curves of GBM devices as shown in Supplementary Fig. S4 . This indicates that the hysteresis of the transfer curve is not caused by the captured molecules, such as a thin layer of water, at the interface of graphene/hBN [23] . Figure 2: Transfer and retention characteristics of heterostructured devices. ( a ) Transfer curve ( I D − V G ) and ( b ) retention performance of the GBM3 device with hBN of 6 nm and MoS 2 of 5 nm. The inset of a shows a transfer curve of GB3. For GBM devices, all the transfer curves in the main text were obtained at V D =100 mV and medium sweep rate of 23 V s −1 . The retention of b was measured at V G =15 V with a pulse of +40 V (red triangle) and −40 V (blue circle), pulse width of 1 ms and V D =100 mV. ( c ) Transfer curve and ( d ) retention performance of the MBG1 device with hBN of 12 nm, MoS 2 of three layers and graphene of two layers. The inset of c shows a transfer curve of the same device when graphene was used for gating. For MBG devices, all the measurement of transfer curve in the main text was obtained at V D =50 mV and medium sweep rate of 23 V s −1 . The retention of d was measured at V G =0 V with pulse of −15 V (violet circle) and +15 V (orange triangle), pulse width of 100 μs and V D =50 mV. Full size image The observed large gate hysteresis can be utilized for a non-volatile memory-device operation employing the MoS 2 layer as a floating gate. The retention of trapped charge by the MoS 2 layer is shown in Fig. 2b . The current ( I D ) in graphene was measured at V G =15 V when gate voltages of ±40 V with pulse width of 1 ms were applied. Two states with different currents can be defined as ‘trap’ and ‘release’ states. The retention performance shows that trapped charge in the MoS 2 layer is maintained without loss of charge. Although I release / I trap is low (~2), most of the GBM devices measured in this work exhibit similar retention characteristics regardless of thicknesses of MoS 2 charge-trap layer and hBN tunnelling barrier. This charge trapping can be preserved over 100 cycles as shown in the endurance characteristic ( Supplementary Fig. S5a ). We observed that even GBM devices with monolayer MoS 2 exhibit charge-trapping characteristics, resulting in large hysteresis and a good trapped charge-retention property ( Supplementary Fig. S6a,b ). Most memory devices relying on charge trapping suffer from problems related to charge retention, such as loss of charge by back-tunnelling, injection of carriers of the opposite type or redistribution of charge in defects [27] . In our multi-stack devices, however, the unique device geometry utilizing a high tunnelling barrier and defect-free crystallinity of 2D crystals provides a solution to circumvent these technical issues. As single-layer graphene has zero band gap, GFETs have an intrinsically small on/off ratio. To overcome this in FET devices, novel design concepts such as graphene barristor have been proposed [28] . For memory devices, a more reasonable solution is the use of 2D material with large band gap. Therefore, we fabricated devices with a reversed stacking order, in which single or multilayer MoS 2 was employed as a channel and graphene was employed as the charge-trapping layer. The transfer curve of the reverse structure MBG1 device exhibited large hysteresis of Δ V ~15 V and high on/off current ratio of 10 4 as shown in Fig. 2c . Similar to GBM devices, different voltage sweep rates showed no appreciable changes in transfer curves of MBG devices as shown in Supplementary Fig. S4d . When graphene was used as a gate electrode, the transfer curve of MBG1 device showed no hysteresis as shown in the inset of Fig. 2c . Moreover, when graphene is grounded, hysteresis of MBG1 device disappeared because of release of the trapped charge from graphene ( Supplementary Fig. S7b,d ). These results demonstrate that the hysteresis of the MBG device is due to charge trapped in the graphene layer rather than at interfaces between the layers. As a result, good retention and endurance were observed ( Fig. 2d and Supplementary Fig. S5b ). High on/off ratio was maintained over 1,400 s. The carrier mobility of MoS 2 in MBG devices ranged from 10 to 40 cm 2 V −1 s −1 , depending on the thickness of MoS 2 . Even though the carrier mobility of MoS 2 is smaller than that of graphene, MBG heterostructure devices should be useful for flexible memory applications requiring the high on/off current ratio. As organic memories are being studied as leading contending devices for future flexible device application, we compared the performances of our GBM and MBG to those of reported organic memories ( Supplementary Table S2 ) [29] , [30] . Compared with organic memories, the heterostructured memory devices fabricated in our study exhibited better performances with advantages of miniaturization, carrier mobility, on/off current ratio, retention and power saving. In addition, the heterostructure memory devices also showed superior stability at high temperature ( Supplementary Figs S8 and S9 ), which implies that these devices can be used in harsh conditions. 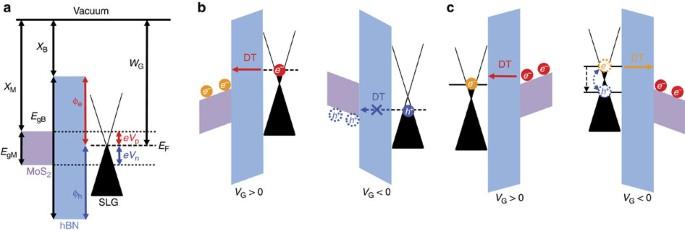Figure 3: Energy band diagram of heterostructured memory devices. Energy band diagrams of (a) flat band state (χ: electron affinity,Eg: band gap,W: work function,ф: tunnelling barrier andeVp(eVn): difference in energy between conduction band (or valence band) of MoS2and Fermi level of graphene;M,B,G,eandhindicate MoS2, hBN, graphene, electron and hole, respectively) and (b) carrier transfer state of GBM device. WhenVG>0 is applied, electrons can be transferred from graphene to MoS2by tunnelling through the hBN barrier. On the other hand, holes in graphene cannot be transferred to MoS2atVG<0. (c) Energy band diagrams of carrier transfer state of MBG device. In trapping process ofVG>0, electrons can be trapped in graphene by tunnelling from MoS2. In releasing process ofVG<0, the trapped electrons in graphene move back to MoS2at initial stage. As the Fermi level of graphene is further reduced and below Dirac point, the trapped electrons can recombine with holes generated in graphene. Effect of charge-trapping layers Figure 3 shows proposed energy band diagrams of the tested devices in the flat band state ( Fig. 3a , with no contact between layers and no applied bias) and in the carrier transfer state ( Fig. 3b ). The work function and electron affinity of MoS 2 are 4.6–4.9 eV and 4.2 eV, respectively [31] , [32] . hBN has larger band gap (5.2–5.9 eV) and smaller electron affinity (2–2.3 eV) [7] , [33] . Thererefore, the barrier heights for electron and hole tunnelling through hBN ( Φ e and Φ h ) are 2.3–2.6 eV and 2.7–3.4 eV, respectively. The work function of a charge-neutral monolayer graphene is 4.6 eV, and it can be further tuned by external electric field [34] . In the case of GBM, when graphene is influenced by electrical field, carrier density in graphene can be calculated by n = C ox / e ( V G − V 0 ), where C ox and e are capacitance of oxide layer and charge of electron, and V 0 is the gate voltage corresponding to the charge neutrality point. The shift of Fermi level can then be expressed by E F = sgn ( n ) ħυ F , where, υ F and ħ are Fermi velocity and Planck’s constant, respectively. With SiO 2 thickness of 280 nm and hBN thickness of 10 nm, C ox / e ~7.5 × 10 10 cm −2 V −1 is obtained. For the gate voltages of −40 V and +40 V in GBM3, the calculated Fermi level shifts of single-layer grapheme (SLG) ( E F ) are −0.19 eV and +0.22 eV, respectively. For this, proximity in energy to conduction ( eV p ) or valence band ( eV n ) of MoS 2 should be considered, because tunnelling probability increases with a line-up of energy states in MoS 2 and graphene. Although these Fermi level shifts can lower the barrier height for tunnelling ( Fig. 3b ), the resulting tunnel barrier height is still too high for Schottky thermal emission. Therefore, it is inferred that the main mechanism of charge transfer through hBN is via quantum tunnelling, which can occur in oxide layers thinner than 6 nm [27] ( Supplementary Fig. S10 ). At small gate voltage, the tunnelling current exponentially increases with decreasing hBN thickness, leading to increasing charge injection for trapping [7] . This trend is further supported by the experimental observation that the hysteresis of the transfer characteristic curves in GBM and MBG is larger for thinner hBN barriers ( Supplementary Figs. S4 and S11 ). Moreover, the change in Fermi level ( E F ) in graphene alters the shape of barrier more significantly for a thinner tunnelling barrier, increasing tunnelling current through thinner hBN [13] . We also note that the tunnelling injection of carriers can be unipolar as indicated in Fig. 3b , electrons in n-doped graphene can be transferred to MoS 2 for V G > 0, while holes in p-doped graphene can hardly move to MoS 2 for V G < 0. The electron tunnelling behaviour through hBN will be explained in detail later. Although carrier transport in the floating gate MoS 2 cannot be measured directly, it is considered that the transferred electrons into MoS 2 are mobile and stay stably in the conduction band, as the grounded charge-trapping layer of MoS 2 causes no hysteresis ( Supplementary Fig. S7c ), and characteristics of programming and erasing are reproducible as shown in Figs 2 and 4 . In MBG devices, graphene acts as a floating gate, which can trap or eject electrons depending on gate voltage as shown in Fig. 3c . When gate voltage is positive in a trapping process, electrons in MoS 2 can be pulled and transferred to graphene by tunnelling. The transferred electrons (orange color) can be trapped in graphene. When gate voltage becomes negative in a releasing process, the trapped electrons can be transferred to MoS 2 , because the negative gate voltage pushes electrons. The Fermi level of graphene is higher than Dirac point in the initial stage of releasing process, because the trapped electrons occupy the energy states over the Dirac point. As the trapped electrons keep transferring to MoS 2 , the Fermi level of graphene will decrease quickly and become close to the Dirac point. Then, electron-hole recombination probably occurs, resulting in fast removal of the trapped electrons. This also can be supported by the results that trapped charges are released and give rise to no hysteresis when the floating gates are grounded ( Supplementary Fig. S7d ). Figure 3: Energy band diagram of heterostructured memory devices. Energy band diagrams of ( a ) flat band state ( χ : electron affinity, E g : band gap, W : work function, ф : tunnelling barrier and eV p ( eV n ): difference in energy between conduction band (or valence band) of MoS 2 and Fermi level of graphene; M , B , G , e and h indicate MoS 2 , hBN, graphene, electron and hole, respectively) and ( b ) carrier transfer state of GBM device. When V G >0 is applied, electrons can be transferred from graphene to MoS 2 by tunnelling through the hBN barrier. On the other hand, holes in graphene cannot be transferred to MoS 2 at V G <0. ( c ) Energy band diagrams of carrier transfer state of MBG device. In trapping process of V G >0, electrons can be trapped in graphene by tunnelling from MoS 2 . In releasing process of V G <0, the trapped electrons in graphene move back to MoS 2 at initial stage. As the Fermi level of graphene is further reduced and below Dirac point, the trapped electrons can recombine with holes generated in graphene. 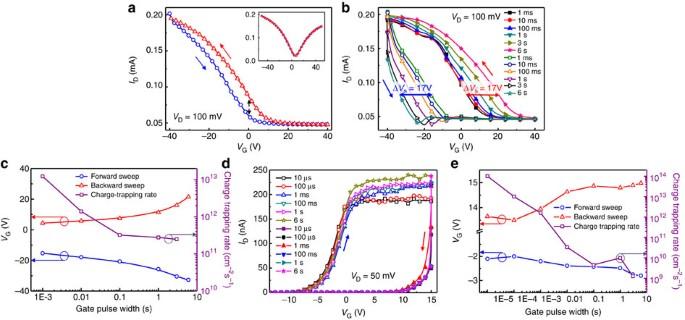Figure 4: Effect of pulse width on transfer characteristics and calculation of charge-trapping rate. (a) Transfer curve of GBM2, which has hBN of 11 nm and MoS2of 3.3 nm. The inset ofashows the transfer curve of GB2 in the same sample. (b) Transfer curves of GBM2 measured with various pulse widths ofVG=±80 V. The filled and blank symbols represent the values measured with +80 V and −80 V, respectively. (c) Gate voltages, which show the sameIDof 78 nA, and calculated charge-trapping rate of GBM2 as a function of gate pulse width. The charge-trapping rate (dNtrap/dt) is estimated by gate shift ΔVSand the pulse width Δt. (d) Transfer curves of MBG1 measured with various pulse widths ofVG=±30 V. The filled and blank symbols represent the values measured with +30 V and −30 V, respectively. (e) Gate voltages, which show the sameIDof 50 nA, and calculated charge-trapping rate of MBG1 as a function of gate pulse width. Full size image Figure 4: Effect of pulse width on transfer characteristics and calculation of charge-trapping rate. ( a ) Transfer curve of GBM2, which has hBN of 11 nm and MoS 2 of 3.3 nm. The inset of a shows the transfer curve of GB2 in the same sample. ( b ) Transfer curves of GBM2 measured with various pulse widths of V G =±80 V. The filled and blank symbols represent the values measured with +80 V and −80 V, respectively. ( c ) Gate voltages, which show the same I D of 78 nA, and calculated charge-trapping rate of GBM2 as a function of gate pulse width. The charge-trapping rate (d N trap /dt) is estimated by gate shift Δ V S and the pulse width Δ t . ( d ) Transfer curves of MBG1 measured with various pulse widths of V G =±30 V. The filled and blank symbols represent the values measured with +30 V and −30 V, respectively. ( e ) Gate voltages, which show the same I D of 50 nA, and calculated charge-trapping rate of MBG1 as a function of gate pulse width. Full size image Charging the floated MoS 2 gate changes the transfer characteristic of the GBM memories significantly. In particular, when a thick MoS 2 layer is used (GBM2), the GFET exhibits a unipolar p-type behaviour, as shown in Fig. 4a . Similar unipolar behaviour was reported in graphene covered with water layer or in doped graphene by metallic oxide, and graphene dual dielectric memory [23] , [35] , [36] . To verify that the unipolar behaviour is due to charge trapping in the MoS 2 layer, we employed two devices fabricated on a same graphene flake without MoS 2 -trapping layer, but one on hBN (GB2) and the other on SiO 2 (GS2) ( Supplementary Fig. S12a ). As seen in inset of Fig. 4a , ambipolar behaviour without hysteresis was observed in GB2 (device without MoS 2 layer). On the other hand, GS2 (device without hBN substrate nor MoS 2 ) exhibits moderate hysteresis (shift less than 5 V), presumably due to adsorbed molecules and charge impurities in SiO 2 (ref. 23 ), but the behaviour remains strongly ambipolar ( Supplementary Fig. S12b ), indicating that the amount of trapped charge is not significant compared with the MoS 2 floating gate. For the thick hBN barrier of 11 nm, the memory operation is also poor. As shown in Fig. 4b , although the hysteresis in p-type GFET operation can be utilized for memory operation, the on/off current ratio was smaller than that obtained using more optimized heterostacks demonstrated in Fig. 2 (GBM3). Similarly, the thicknesses of hBN and graphene in MBG devices influence the FET performance (see Supplementary Fig. S11 ). When the thicknesses of the tunnel barrier of hBN and charge-trapping layer of graphene are reduced, larger hysteresis and higher on/off current ratio are observed. This is because larger amount of charge can tunnel through thinner hBN and the electric field by a gate voltage is more weakly screened by thinner graphene [7] , [13] , [37] . We now discuss a potential source of the asymmetric gate characteristics with the MoS 2 floating gate. The asymmetry of the observed hysteresis suggests that tunnelling of electrons and holes at positive and negative gate voltages is asymmetric. This asymmetry can be due to different tunnel barrier heights for electrons and holes [13] , or a larger effective mass of holes ( m h =0.5 m 0 ) than electrons ( m e =0.26 m 0 ) in hBN [38] . A large electron tunnelling probability [39] can lead to a gate-independent channel current at positive gate voltages, as shown in GBM2 and GBM3; electrons in the graphene tunnel rapidly into the MoS 2 trap layer and then screen the electric field from the back gate to reach the graphene channel, whereas the low possibility of hole-tunnelling process does not provide enough charge for screening. This effect is not seen in GBM1, with monolayer MoS 2 ( Supplementary Fig. S4a ); in such a device with very thin MoS 2 -trapping layers, the amount of trapped charges might not be enough to provide sufficient gate-field screening. The larger hysteresis observed in GBM3 than that in GBM2 ( Supplementary Fig. S4b,c ) is because of the thinner hBN tunnelling layer and thicker MoS 2 -trapping layer in GBM3, which induces larger electron tunnelling current providing better screening. We now discuss the dynamic transition rate of floating gate devices. For this purpose, we pulse the gate and measure the transfer characteristics to estimate the trapping and detrapping rates of the charge into and from the charge-trapping layer. Figure 4b shows the hysteresis of device GBM2 as a function of gate pulse width. Here the gate pulses of ±80 V were applied, with the varying pulse width in the range of 1 ms–6 s followed by the transfer curve measurement. The transfer characteristics are measured as reverse sweeps (+40 to −40 V) following +80 V gate pulses, and forward sweeps (−40 to +40 V) following −80 V gate pulses. The transfer curve hysteresis loop widens with increasing pulse width up to 6 s, and saturates after that ( Fig. 4b ). As the saturated gate voltage shift (Δ V s ) is ~17 V, charge-trap density is estimated to be N = C ox Δ V s / e ~1.28 × 10 12 cm −2 , which is larger than a typical trap-charge density of 2.5 × 10 11 cm −2 in SiO 2 (ref. 40 ). The electron trapping rate in MoS 2 (or, equivalently, the hole-releasing rate from MoS 2 ) is then estimated from (d N trap /dt)=( C ox / e ) (d V G /d t ) by using d V G /d t ~Δ V s /Δ t , where Δ t is the pulse width and Δ V s is the gate voltage shift. Figure 4c shows both Δ V s and charge-trapping rate as a function of gate pulse width. The charge-trapping rate (d N trap /d t ) varies from 10 13 to 10 11 cm −2 s −1 as the pulse width changes from 1 ms to 6 s, indicating the energy level of the trap sites may differ considerably. We also note that the charge-trapping rate is relatively fast compared with a typical value, ~10 9 cm −2 s −1 , in metal–insulator–semiconductor [41] . Separating from the trapping rate, the charge-transfer rate, d N transfer /d t , governed by the tunnelling process, can be estimated from the tunnelling current. In principle, the charge-transfer rate can be expressed by d N transfer /d t=I tunnel / Ae , where I tunnel , A and e are tunnel current, device area and electric charge, respectively. Although we have not monitored the gate tunnelling current, we can utilize the tunnelling measurement result across an hBN layer of similar thickness (see Supplementary Fig. S10 ), where a charge-transfer rate of 1.18 × 10 13 cm −2 s −1 is estimated. Note that this value is similar to the charge-trapping rate for the short period of pulse <1 ms, but larger for the longer period of pulse shown in Fig. 4c . This suggests that trapping dynamic control is more important than the tunnelling process control for fast memory operation at this point. We believe that this charge-trapping rate can be further enhanced by optimizing the thickness of hBN and MoS 2 layers, so that Δ V can be enlarged to be more suitable for faster memory device application. Figure 4d shows transfer curves of MBG1 measured with various pulse widths of V G =±30 V. Both Δ V s and charge-trapping rate as a function of gate pulse width are shown in Fig. 4e . The MBG device showed the reasonable memory window even at short pulse width of 10 μs. The charge-trapping rate varies from 10 14 to 10 9 cm −2 s −1 . It should be noted that charge-trapping rate at the same pulse width is slower compared with GBM devices. As the thickness of hBN used in MBG and GBM devices here is similar, the difference in charge-trapping rate is attributed to the smaller density of states in the MBG device compared with the GBM device. We studied the charge-trapping characteristics of MoS 2 and graphene in multi-stacked graphene/hBN/MoS 2 (GBM) and MoS 2 /hBN/graphene (MBG) devices. GBM devices on the stacked hBN/MoS 2 showed different hysteresis characteristics, depending on the thicknesses of MoS 2 and hBN. From the measurement of retention and endurance characteristics, it was confirmed that the MoS 2 layer acts as an effective charge-trapping layer. When thicker MoS 2 layer and thinner hBN were employed, unipolar conductance and larger hysteresis were observed because of effective electron tunnelling and electric-field screening. Meanwhile, when the reversed stacking structure of MBG was investigated, high on/off current ratio and large memory window were attained. This study provides a promising route of future flexible and transparent memory device operation, utilizing ultrathin and flexible 2D materials. Device fabrication Heterostructured devices were fabricated by stacking 2D materials. For GBM devices, thin layers of MoS 2 were mechanically exfoliated on a silicon wafer with 280-nm-thick SiO 2 . After hBN and SLG were exfoliated onto wafers coated with polymethyl methacrylate (PMMA) and a thin release layer, PMMA film was removed from the wafer, then hBN and SLG were sequentially transferred onto the wafer containing the MoS 2 , as reported previously [4] , [13] (see Supplementary Fig. S1 ). MBG devices were fabricated by a similar method, in a reverse-stacking order. For removal of PMMA residues generated during the stacking process, the samples were annealed at 345 °C by flowing H 2 /Ar-forming gas between transfer steps [4] , [13] . Source and drain electrodes were patterned using electron-beam lithography and deposition of Cr/Pd/Au (1/10/50 nm) for GBM and Ti/Au (0.5/50 nm) for MBG, where the doped Si substrate underneath the SiO 2 layer was used as a back gate. To verify the effect of charge-trapping layer, two devices with or without charge-trapping layer are fabricated by an additional electron-beam lithography process followed by oxygen plasma etching. Characterization of materials Atomic force microscopy (Park Systems, XE-100) and Raman spectroscopy (Renishaw, inVia) were used to ensure the qualities and thicknesses of graphene, hBN and MoS 2 . The laser of 532 nm wavelength was used for the excitation in Raman spectroscopy. Even though Raman spectra of MoS 2 covered by hBN are not sharp as shown in Supplementary Fig. S2a , the separation between two peaks indicate the number of layers. To check the quality of MoS 2 , hBN and graphene, therefore, the exfoliated flakes were tested using Raman spectroscopy and micro-PL spectroscopy before the transfer steps as shown in Supplementary Fig. S2b–d . It is difficult to estimate the defect density in graphene sitting on hBN, because the D peak of graphene and the main peak of hBN are located at the same position of 1,370 cm −1 ( Supplementary Fig. S2d ) [42] . As shown in Supplementary Fig. S2a,b , MoS 2 flakes with various thicknesses showed different peak separations and PL intensities as reported [6] , [43] . The narrow width (~80 meV) of PL peak around 1.84 eV indicates that MoS 2 has high crystallinity [6] . Electrical characterization of devices Electrical properties of fabricated devices were measured with a semiconductor parameter analyzer (Agilent, 4155C) in vacuum and at room temperature. The fabricated GBM and MBG devices showed high mobilities of graphene (~4,200 cm 2 V −1 s −1 ) and MoS 2 (~35 cm 2 V −1 s −1 for three layers). For measurement of tunnelling current through hBN, a simple metal–insulator–metal device was fabricated as shown in Supplementary Fig. S10a . To make a flat bottom electrode, a pristine few-layer graphene was used. The breakdown voltage for Fowler–Nordheim tunnelling in this device is ~6 V (6 MV cm −1 ), which corresponds to the electric field of 180 V when using Si back gate in a Si substrate with 300-nm-thick SiO 2 . This indicates that, because back gate voltage of 40 V was used in the GBM devices, the Fowler–Nordheim tunnelling does not take place in the devices. Even though the dielectric strength in this device is smaller than the reported value (8 MV cm −1 ; ref. 7 ), high-temperature treatment-like annealing process can lower the dielectric strength of hBN by generating defects [44] . As the annealing temperature increases, tunnelling current through hBN was enhanced probably by trap-assisted tunnelling. As shown in Supplementary Fig. S10b , tunnelling current through hBN slightly increases with temperature. However, tunnelling was not affected by exposure of light (100 W) as shown in Supplementary Fig. S10c . Measurement of temperature dependence To clarify the effect of temperature on tunnelling and charge trapping, transfer curves of the GBM4 and MBG3 devices were obtained at different temperature as shown in Supplementary Fig. S8 . For GBM4 device, even though a small decrease in on-current, maybe due to thermal disturbance, was observed, large hysteresis was maintained at 200 °C. It is estimated that the larger memory window and two charge-neutral points at both negative- and positive-gate voltages are attributed to p-doping of graphene during the fabrication process. In contrast, the MBG3 device exhibited no significant temperature dependence as shown in Supplementary Fig. S8b . The small increase in hysteresis and on-current are probably due to thermal excitation to overcome the contact barrier between MoS 2 and metal electrode. As shown in Supplementary Fig. S9 , there is no appreciable difference in retention performance of the MBG3 device even at 200 °C. The trapped charge can be released by back-tunnelling, and tunnelling can be assisted by high temperature. However, our result indicates that the trapped charge can be stored efficiently without any loss. Therefore, it is evident that the heterostructure memory devices suggested in this study are stable at high temperature; therefore, it can be applied in the harsh conditions. How to cite this article: Choi, M. S. et al . Controlled charge trapping by molybdenum disulphide and graphene in ultrathin heterostructured memory devices. Nat. Commun. 4:1624 doi: 10.1038/ncomms2652 (2013).